Opposing regulation of dopaminergic activity and exploratory motor behavior by forebrain and brainstem cholinergic circuits Dopamine transmission is critical for exploratory motor behaviour. A key regulator is acetylcholine; forebrain acetylcholine regulates striatal dopamine release, whereas brainstem cholinergic inputs regulate the transition of dopamine neurons from tonic to burst firing modes. How these sources of cholinergic activity combine to control dopamine efflux and exploratory motor behaviour is unclear. Here we show that mice lacking total forebrain acetylcholine exhibit enhanced frequency-dependent striatal dopamine release and are hyperactive in a novel environment, whereas mice lacking rostral brainstem acetylcholine are hypoactive. Exploratory motor behaviour is normalized by the removal of both cholinergic sources. Involvement of dopamine in the exploratory motor phenotypes observed in these mutants is indicated by their altered sensitivity to the dopamine D2 receptor antagonist raclopride. These results support a model in which forebrain and brainstem cholinergic systems act in tandem to regulate striatal dopamine signalling for proper control of motor activity. Dopamine (DA) transmission has been implicated in a variety of motor, emotional and cognitive functions [1] , [2] , [3] . Midbrain DA neurons in the substantia nigra pars compacta (SNc) and ventral tegmental area (VTA) provide important modulatory input to the striatal complex, including the caudate putamen (CPu) and nucleus accumbens (NAc). Acetylcholine (ACh) signalling pathways regulate DA efflux within the striatum at two fundamental levels of the circuit [4] . First, the burst firing of DA neurons in the SNc and VTA is stimulated perisomatically by glutamatergic and cholinergic inputs from the pedunculopontine tegmental (PTg) and laterodorsal tegmental (LDTg) nuclei in the rostral brainstem [5] , [6] , [7] , thereby resulting in increased striatal DA efflux [6] and locomotor activity [8] . In particular, cholinergic inputs from the LDTg appear to act as a gate for the transition from tonic to burst firing modes, thereby regulating the responsiveness of DA neurons to glutamatergic signalling [9] . Second, ACh release from striatal cholinergic interneurons can trigger DA release via presynaptic nicotinic ACh receptors (nAChRs) on DA axons [10] , [11] , [12] . Inhibition or desensitization of nAChRs on DAergic axons in striatal slices leads to a decrease in DA release evoked by a single stimulus pulse, but an increase in release evoked at burst-like frequencies, thus amplifying the frequency dependence of axonal DA release as monitored by fast-scan cyclic voltammetry [13] , [14] . Although striatal ACh can also affect the excitability of medium spiny neurons directly by signalling through muscarinic ACh receptors (mAChRs) [15] , intrastriatal injections of scopolamine, a mAChR antagonist, does not alter motor activity [16] . In addition to local cholinergic regulation of DA efflux within the striatum, ACh arising from projection neurons within the ventral forebrain (for example, nucleus basalis of Meynert) likely regulates striatal DA efflux indirectly via modulation of descending glutamatergic pathways from the prefrontal cortex, ventral pallidum and hippocampus to the SNc/VTA [17] , [18] . Thus, we hypothesized that broad removal of ACh within the forebrain would result in exaggerated striatal DA signalling and altered motor behaviours in a manner dependent on the stimulation of burst firing of midbrain DA neurons by brainstem-derived ACh. To test the relative contributions of forebrain and brainstem cholinergic input to the regulation of DAergic activity, we took advantage of genetic ablation strategies in mice to eliminate ACh synthesis selectively in the forebrain, brainstem, or both regions simultaneously. We then assessed the effects on evoked striatal DA release in vitro , and the behavioural propensity for open field exploration when placed in a novel environment, which is highly responsive to changes in striatal DA efflux [19] , [20] . We found that mice lacking forebrain ACh showed enhanced phasic-to-tonic DA release throughout the striatal complex, and exhibited locomotor hyperactivity in a novel environment. By contrast, exploratory motor behaviour was reduced in mice lacking brainstem ACh, consistent with a predicted decrease in DA neuron burst firing, with lower striatal DA signalling indicated by a lack of sensitivity to the DA D2 receptor antagonist raclopride. Remarkably, exploratory motor behaviour was normalized in mice lacking both forebrain and brainstem ACh. These findings highlight the critical roles that forebrain and brainstem cholinergic systems have in driving striatal DAergic activity for the control of exploratory motor activity. Generation of forebrain ACh knockout mice The enzyme choline acetyltransferase (ChAT) is essential for ACh synthesis. To generate animals with a forebrain-restricted ablation of ACh production, we combined a conditional floxed allele of ChAT ( ChAT flox ) [21] with an Nkx2.1 Cre transgenic line in which cumulative recombination is restricted to the forebrain and hypothalamus [22] ( Fig. 1a ). Using an antisense cRNA probe directed against the floxed exons, we performed in situ hybridization for ChAT mRNA on cryosections prepared from non-mutant transgenic control (see Methods) and ChAT forebrain knockout (KO; Nkx2.1 Cre ; ChAT flox/flox ; ‘forebrain KO’) brains at P30. These analyses revealed almost complete elimination of ChAT expression from striatal cholinergic interneurons, with only 6±3 ChAT -positive cells in a representative set of forebrain KO striatal sections that spanned the rostrocaudal extent of the striatum (seven sections from each of three brains) versus 442±18 ChAT -positive cells in comparable sections from control brains (seven sections from each of three brains) ( Fig. 1c ). Similar efficacy of ChAT removal was also observed in the medial septum, diagonal band and nucleus basalis ( Fig. 1e ); cortical cholinergic interneurons were not affected as this VIP + population does not arise from an Nkx2.1 expressing lineage [22] . Importantly, Nkx2.1 Cre does not affect ChAT expression in the brainstem of ChAT flox/flox animals ( Fig. 1g ). 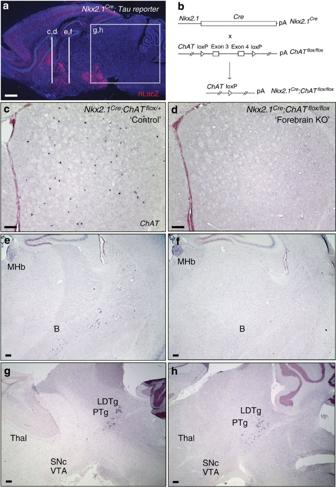Figure 1: Genetic strategies for targeted ablation of ACh production in the forebrain. (a) Sagittal field of a P21Nkx2.1Cre;TauloxP-stop-loxP-mGFPiresNLSLacZ(‘Tau reporter’) mouse brain illustrating the populations (nLacZ+; red) that arise fromNkx2.1 expressing lineages. (b) Genetic strategy for selective elimination of ACh production within the forebrain (Nkx2.1lineages). (c,d)In situhybridization forChATmRNA in coronal striatal brain cryosections fromNkx2.1Cre; ChATflox/+non-mutant control (c) andNkx2.1Cre; ChATflox/floxforebrain KO (d) mice at P30 revealed a complete loss ofChATexpression in the striatum of the forebrain KO. (e,f) Coronal fields of control (Nkx2.1Cre; ChATflox/+;e) and mutant (‘forebrain KO’;Nkx2.1Cre; ChATflox/flox;f) P30 brain sections stained byin situhybridization forChATmRNA illustrate the removal ofChATexpression within the nucleus basalis, in addition to the striatum (c,d) and other ventral forebrain cholinergic populations. (g,h)ChATexpression within the rostral brainstem (for example, PTg, LDTg) is not affected in the forebrain KO. Scale bar inarepresents 1 mm; scale bars inc–hrepresent 300 μm. B, nucleus basalis of Meynert; LDTg, laterodorsal tegmental nucleus; MHb, medial habenular nucleus; PTg, pedunculopontine nucleus; Thal, thalamus; VTA, ventral tegmental area. Figure 1: Genetic strategies for targeted ablation of ACh production in the forebrain. ( a ) Sagittal field of a P21 Nkx2.1 Cre ; Tau loxP-stop-loxP-mGFPiresNLSLacZ (‘ Tau reporter ’) mouse brain illustrating the populations (nLacZ + ; red) that arise from Nkx2. 1 expressing lineages. ( b ) Genetic strategy for selective elimination of ACh production within the forebrain ( Nkx2.1 lineages). ( c , d ) In situ hybridization for ChAT mRNA in coronal striatal brain cryosections from Nkx2.1 Cre ; ChAT flox/+ non-mutant control ( c ) and Nkx2.1 Cre ; ChAT flox/flox forebrain KO ( d ) mice at P30 revealed a complete loss of ChAT expression in the striatum of the forebrain KO. ( e , f ) Coronal fields of control ( Nkx2.1 Cre ; ChAT flox/+ ; e ) and mutant (‘forebrain KO’; Nkx2.1 Cre ; ChAT flox/flox ; f ) P30 brain sections stained by in situ hybridization for ChAT mRNA illustrate the removal of ChAT expression within the nucleus basalis, in addition to the striatum ( c , d ) and other ventral forebrain cholinergic populations. ( g , h ) ChAT expression within the rostral brainstem (for example, PTg, LDTg) is not affected in the forebrain KO. Scale bar in a represents 1 mm; scale bars in c – h represent 300 μm. B, nucleus basalis of Meynert; LDTg, laterodorsal tegmental nucleus; MHb, medial habenular nucleus; PTg, pedunculopontine nucleus; Thal, thalamus; VTA, ventral tegmental area. Full size image Increased phasic-to-tonic DA release in forebrain ACh KO mice We next examined the consequences of loss of forebrain cholinergic transmission on local DA release regulation using fast-scan cyclic voltammetry to monitor evoked extracellular DA concentration ([DA] o ) in the dorsolateral region of the CPu in striatal slices. Release was evoked by either a single-pulse (1 p) stimulation that mimics one action potential or by brief five-pulse (5 p), phasic stimulation at varying frequencies. Consistent with previous pharmacological evidence that endogenous striatal ACh facilitates tonic DA release [13] , [14] , peak [DA] o evoked by 1 p or by 5 p at low frequencies (≤10 Hz) was decreased in forebrain KO slices compared with control slices ( Fig. 2a ). However, peak [DA] o evoked by high frequency (100 Hz) stimulation was dramatically higher in the forebrain KO CPu ( Fig. 2a ). To establish whether the contrast between phasic-to-tonic DA release differed in control versus forebrain KO mice, we determined the ratio of 5 p evoked [DA] o to that evoked by 1 p at individual DA release sites; comparison of 5 p-to-1 p ratios also normalized differences in absolute evoked [DA] o between recording sites. These data revealed a marked frequency dependence of DA release in the forebrain KO CPu that was absent in slices from control animals ( P <0.001 at 25, 50 and 100 Hz in forebrain KO versus control, two-way analysis of variance (ANOVA), Bonferroni correction, n =16–18 recording sites from four to five mice per group) ( Fig. 2c ). The pattern of increased frequency responsiveness of DA release mirrored that seen in control slices when nAChRs were blocked by mecamylamine (5 μM) or desensitized by nicotine (500 nM) ( Fig. 2c ). Moreover, in contrast to the effects seen in control slices, neither mecamylamine nor nicotine had a significant effect on [DA] o evoked by either tonic or phasic (>10 Hz) stimulation ( Fig. 2c ), demonstrating the complete absence of nAChR-dependent regulation of DA release in the CPu of forebrain KO animals. 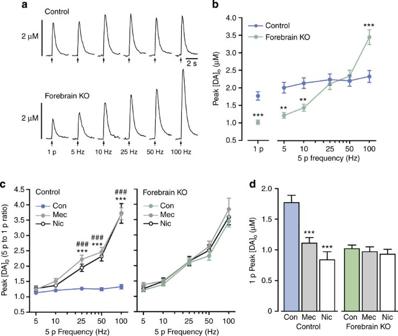Figure 2: Loss of forebrain ACh production results in enhanced phasic-to-tonic DA signalling within the dorsal striatum. (a–d) Voltammetric monitoring of extracellular [DA]oin the CPu of striatal slices. (a) Representative single-pulse (1 p) and five-pulse (5 p) evoked [DA]orecorded in control and forebrain KO mice. (b) Mean peak [DA]oevoked by 1 p and 5 p stimulation in each group shows suppression of DA release up to 10 Hz, maintenance of release levels at 25 and 50 Hz, and enhanced peak [DA]oat 100 Hz (**P<0.01; ***P<0.001 versus control; unpairedt-test for comparison of 1 p or two-way ANOVA with Bonferroni correction for comparison of 5 p). (c) Frequency dependence (5 p-to-1 p ratio) of evoked [DA]oin control and forebrain KO mice under control conditions (con) and in the presence of the nAChR antagonist mecamylamine (mec; 5 μM) or a desensitizing concentration of the nAChR agonist nicotine (nic; 500 nM) (***P<0.001 mec versus con,###P<0.001 nic versus con, two-way ANOVA with Bonferroni correction). The 1 p-to-5 p ratios in forebrain KO mice under control conditions were indistinguishable from those in control mice in mec or nic (P>0.05 for each frequency for either mec or nic, two-way ANOVA with Bonferroni correction). (d) 1 p evoked [DA]oin forebrain KO mice, unlike in control mice, was not suppressed by either mec or nic (***P<0.001 versus con, one-way ANOVA with Dunnett’s correction). Control data are from four mice withn=16 recording sites in control conditions andn=8 sites in each drug. Data for forebrain KOs are from five mice withn=18 recording sites in control conditions andn=9 sites in each drug. All data are means±s.e.m. con, control conditions; mec, mecamylamine; nic, nicotine. Figure 2: Loss of forebrain ACh production results in enhanced phasic-to-tonic DA signalling within the dorsal striatum. ( a – d ) Voltammetric monitoring of extracellular [DA] o in the CPu of striatal slices. ( a ) Representative single-pulse (1 p) and five-pulse (5 p) evoked [DA] o recorded in control and forebrain KO mice. ( b ) Mean peak [DA] o evoked by 1 p and 5 p stimulation in each group shows suppression of DA release up to 10 Hz, maintenance of release levels at 25 and 50 Hz, and enhanced peak [DA] o at 100 Hz (** P <0.01; *** P <0.001 versus control; unpaired t -test for comparison of 1 p or two-way ANOVA with Bonferroni correction for comparison of 5 p). ( c ) Frequency dependence (5 p-to-1 p ratio) of evoked [DA] o in control and forebrain KO mice under control conditions (con) and in the presence of the nAChR antagonist mecamylamine (mec; 5 μM) or a desensitizing concentration of the nAChR agonist nicotine (nic; 500 nM) (*** P <0.001 mec versus con, ### P <0.001 nic versus con, two-way ANOVA with Bonferroni correction). The 1 p-to-5 p ratios in forebrain KO mice under control conditions were indistinguishable from those in control mice in mec or nic ( P >0.05 for each frequency for either mec or nic, two-way ANOVA with Bonferroni correction). ( d ) 1 p evoked [DA] o in forebrain KO mice, unlike in control mice, was not suppressed by either mec or nic (*** P <0.001 versus con, one-way ANOVA with Dunnett’s correction). Control data are from four mice with n =16 recording sites in control conditions and n =8 sites in each drug. Data for forebrain KOs are from five mice with n =18 recording sites in control conditions and n =9 sites in each drug. All data are means±s.e.m. con, control conditions; mec, mecamylamine; nic, nicotine. Full size image Given differential regulation of DA release in dorsal and ventral striatum by ACh acting at nAChRs and mAChRs [23] , [24] , [25] , we examined patterns of evoked [DA] o in the NAc core and shell to address whether enhancement in phasic-to-tonic DA signalling in forebrain KO mice occurred throughout the dorsoventral extent of the striatal complex. Peak evoked [DA] o by 1 p was lower in NAc core and shell than in CPu in control mice, with CPu >NAc core >NAc shell ( P <0.001 CPu versus NAc shell, one-way ANOVA, Bonferroni correction, n =16 sites from four mice for CPu, n =9 sites from three mice for NAc core and shell). Also differing from CPu, both NAc core and shell exhibited bell-shaped frequency response curves with 5 p stimulation ( Fig. 3 ), as reported previously [23] , [24] , [26] , [27] . Nevertheless, DA release evoked by 1 p or low-frequency 5 p stimulation was lower than in control mice in the NAc of forebrain KO mice ( Fig. 3a ). By contrast, release evoked by high frequency stimulation was enhanced in both NAc subregions of forebrain KO mice ( Fig. 3a ), resulting in a marked amplification of phasic-to-tonic DA signalling at frequencies >10 Hz ( P <0.001 at 25, 50 and 100 Hz in forebrain KO versus control, two-way ANOVA, Bonferroni correction, n =9–14 recording sites from three mice per group) ( Fig. 3a ). These data confirm the loss of DA release regulation by endogenous ACh throughout the striatal complex of forebrain KO mice. 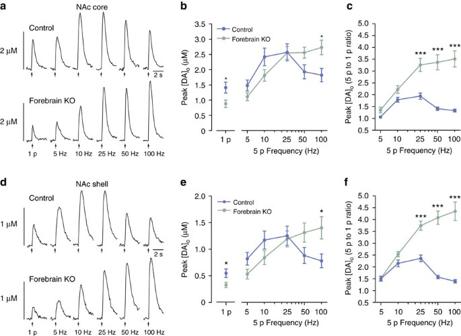Figure 3: Loss of forebrain Ach production results in enhanced phasic-to-tonic DA signalling within the ventral striatum. (a–f) Voltammetric monitoring of extracellular [DA]oin the NAc of striatal slices. (a,d) Representative single-pulse (1 p) and five-pulse (5 p) evoked [DA]orecorded in non-mutant control and forebrain KO mice in the NAc core (a) and NAc shell (d). (b,e) Mean peak [DA]oevoked by 1 p and 5 p stimulation in each group shows suppression of DA release up to 10 Hz (*P<0.05 versus control for 1p; unpairedt-test or two-way ANOVA with Bonferroni correction for comparison of 5 p), maintenance of release levels at 25 Hz and enhanced peak [DA]oat 50 and 100 Hz (*P<0.05 versus control for 100 Hz; two-way ANOVA with Bonferroni correction) in both the NAc core (b) and NAc shell (e). (c,f) Frequency dependence (5 p-to-1 p ratio) of evoked [DA]oin control and forebrain KO mice under control conditions. The 1 p-to-5 p ratios in forebrain KO mice were enhanced at frequencies above 25 Hz (***P<0.001 for each frequency, two-way ANOVA with Bonferroni correction) in both the NAc core (c) and NAc shell (f) indicating enhanced phasic-to-tonic DA signalling throughout the ventral striatum with loss of ACh. Data for NAc core are from three control mice and three forebrain KOs withn=14 recording sites in each. Data for NAc shell are from three control mice withn=9 recording sites and three forebrain KOs withn=11 recording sites. All data are means±s.e.m. Figure 3: Loss of forebrain Ach production results in enhanced phasic-to-tonic DA signalling within the ventral striatum. ( a – f ) Voltammetric monitoring of extracellular [DA] o in the NAc of striatal slices. ( a , d ) Representative single-pulse (1 p) and five-pulse (5 p) evoked [DA] o recorded in non-mutant control and forebrain KO mice in the NAc core ( a ) and NAc shell ( d ). ( b , e ) Mean peak [DA] o evoked by 1 p and 5 p stimulation in each group shows suppression of DA release up to 10 Hz (* P <0.05 versus control for 1p; unpaired t -test or two-way ANOVA with Bonferroni correction for comparison of 5 p), maintenance of release levels at 25 Hz and enhanced peak [DA] o at 50 and 100 Hz (* P <0.05 versus control for 100 Hz; two-way ANOVA with Bonferroni correction) in both the NAc core ( b ) and NAc shell ( e ). ( c , f ) Frequency dependence (5 p-to-1 p ratio) of evoked [DA] o in control and forebrain KO mice under control conditions. The 1 p-to-5 p ratios in forebrain KO mice were enhanced at frequencies above 25 Hz (*** P <0.001 for each frequency, two-way ANOVA with Bonferroni correction) in both the NAc core ( c ) and NAc shell ( f ) indicating enhanced phasic-to-tonic DA signalling throughout the ventral striatum with loss of ACh. Data for NAc core are from three control mice and three forebrain KOs with n =14 recording sites in each. Data for NAc shell are from three control mice with n =9 recording sites and three forebrain KOs with n =11 recording sites. All data are means±s.e.m. Full size image Generating brainstem and double forebrain/brainstem ACh KO mice Using a similar genetic approach to that used to produce forebrain ChAT KO mice, we generated rostral brainstem ChAT KO animals using the En1 Cre driver [28] , whose cumulative recombination is restricted to the mes/r1 embryonic territory ( Fig. 4a ), and as such, primarily affects the PTg and LDTg but not brainstem motor nuclei that arise from more caudal regions (for example, Mo5) ( Fig. 4c ). ChAT brainstem KO mice ( En1 Cre ; ChAT flox/flox ; ‘brainstem KO’) had no ChAT -positive cells remaining in the rostral brainstem as determined by in situ hybridization in a representative set of sections, whereas control mice had 234±10 ChAT -positive cells in comparable fields ( n =3 brains for each genotype, five comparable sections spanning the PTg/LDTg region counted per brain) ( Fig. 4c ). Demonstrating the regional segregation of this ablation strategy, striatal ChAT expression in brainstem KO mice did not differ from that in control mice ( Fig. 4e ). We then combined these two conditional KO strategies and generated forebrain/brainstem ACh ‘double KO’ mice. 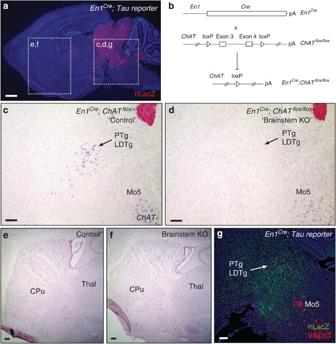Figure 4: Genetic strategies for targeted ablation of ACh production in the rostral brainstem. (a) Sagittal field of a P21En1Cre; TauloxP-stop-loxP-mGFPiresNLSLacZ(‘Tau reporter’) mouse brain illustrating the populations (nLacZ+; red) that arise fromEn1expressing lineages. (b) Genetic strategy for selective elimination of ACh production within the rostral brainstem (En1lineages). (c,d)In situhybridization forChATmRNA in sagittal brainstem cryosections fromEn1Cre; ChATflox/+non-mutant control (c) andEn1Cre; ChATflox/floxbrainstem KO (d) mice at P30 revealed a complete loss ofChATexpression in the PTg/LDTg of the brainstem KO, but normalChATexpression in Mo5. (e,f) Sagittal fields of control (En1Cre; ChATflox/+;e) and mutant (‘brainstem KO’;En1Cre; ChATflox/flox;f) P30 forebrain sections stained byin situhybridization forChATmRNA reveals normalChATexpression in the forebrain of brainstem KO mice. (g) Sagittal field of a P21En1Cre; Tau reporterbrain section stained by immunohistochemistry for nuclear β-galactosidase (nLacZ; green) and vesicular acetylcholine transporter (VAChT; red) reveals complete labelling of the PTg/LDTg but no labelling within Mo5. Scale bar inarepresents 1 mm; scale bars inc–grepresent 300 μm. CPu, caudate putamen; LDTg, laterodorsal tegmental nucleus; Mo5, motor trigeminal nucleus; PTg, pedunculopontine nucleus; Thal, thalamus. Figure 4: Genetic strategies for targeted ablation of ACh production in the rostral brainstem. ( a ) Sagittal field of a P21 En1 Cre ; Tau loxP-stop-loxP-mGFPiresNLSLacZ (‘ Tau reporter ’) mouse brain illustrating the populations (nLacZ + ; red) that arise from En1 expressing lineages. ( b ) Genetic strategy for selective elimination of ACh production within the rostral brainstem ( En1 lineages). ( c , d ) In situ hybridization for ChAT mRNA in sagittal brainstem cryosections from En1 Cre ; ChAT flox/+ non-mutant control ( c ) and En1 Cre ; ChAT flox/flox brainstem KO ( d ) mice at P30 revealed a complete loss of ChAT expression in the PTg/LDTg of the brainstem KO, but normal ChAT expression in Mo5. ( e , f ) Sagittal fields of control ( En1 Cre ; ChAT flox/+ ; e ) and mutant (‘brainstem KO’; En1 Cre ; ChAT flox/flox ; f ) P30 forebrain sections stained by in situ hybridization for ChAT mRNA reveals normal ChAT expression in the forebrain of brainstem KO mice. ( g ) Sagittal field of a P21 En1 Cre ; Tau reporter brain section stained by immunohistochemistry for nuclear β-galactosidase (nLacZ; green) and vesicular acetylcholine transporter (VAChT; red) reveals complete labelling of the PTg/LDTg but no labelling within Mo5. Scale bar in a represents 1 mm; scale bars in c – g represent 300 μm. CPu, caudate putamen; LDTg, laterodorsal tegmental nucleus; Mo5, motor trigeminal nucleus; PTg, pedunculopontine nucleus; Thal, thalamus. Full size image DA release in brainstem and forebrain/brainstem ACh KO mice To confirm that local cholinergic regulation of striatal DA was functionally intact in brainstem KO mice, we examined the frequency dependence of evoked DA release in striatal slices from these animals. Patterns of 1 p and 5 p evoked [DA] o in the CPu of these animals did not differ from those in control mice ( Fig. 5a ), and were as sensitive as controls to nAChR antagonism by mecamylamine or by nicotine-induced desensitization ( Fig. 5c ). These in vitro data demonstrate that there is no alteration in local cholinergic regulation of striatal DA release or other compensatory changes in response to the chronic loss of brainstem ACh. We then examined DA release in striatal slices from double KO mice. As in forebrain KO mice, 1 p evoked [DA] o in the CPu was lower in double KO versus control mice with enhanced phasic-to-tonic DA release, and concomitant loss of effect of mecamylamine and nicotine on evoked [DA] o ( Fig. 5 ). These data confirm the functional loss of forebrain ACh in double KO mice, as seen in forebrain KO mice. Of course, in these in vitro experiments the pattern of stimulation is experimenter driven, whereas in vivo the pattern will be determined by DA neuron firing activity that then undergirds striatal DA release [29] and its consequent influence on motor behaviour. 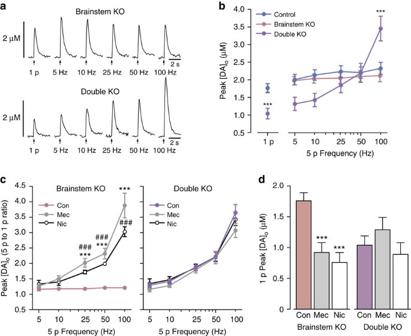Figure 5: Loss of brainstem-derived ACh does not affect local regulation of striatal DA release. (a–d) Voltammetric measurements of extracellular [DA]oin the CPu of striatal slices. (a) Representative single-pulse (1 p) and five-pulse (5 p) evoked [DA]orecorded in brainstem KO and forebrain/brainstem double KO mice. (b,c) Mean peak [DA]oevoked by 1 p and 5 p stimulation shows that DA release is not significantly altered in brainstem KO versus control mice (b). In double KO mice, there is a general suppression of DA release up to 10 Hz, maintenance of release levels at 25 and 50 Hz, and enhanced peak [DA]oat 100 Hz (b) (***P<0.001 versus control; unpairedt-test for comparison of 1 p or two-way ANOVA with Bonferroni correction for comparison of 5 p). (c) Frequency dependence (5 p-to-1 p ratio) of evoked [DA]oin brainstem and double KO mice under control conditions (con) and in the presence of the nAChR antagonist mecamylamine (mec; 5 μM) or a desensitizing concentration of the nAChR agonist nicotine (nic; 500 nM) (***P<0.001 mec versus con,###P<0.001 nic versus con, two-way ANOVA with Bonferroni correction). The 1 p-to-5 p ratio in double KO mice under control conditions was indistinguishable from those seen in control mice in mec or nic (P>0.05 for each frequency for either mec or nic, two-way ANOVA with Bonferroni correction). (d) 1 p evoked [DA]oin double KO mice was not suppressed by either mec or nic, in contrast to brainstem KO mice (***P<0.001 versus con, one-way ANOVA with Dunnett’s correction). Data for brainstem KOs are derived from four mice withn=16 recording sites in con andn=8 sites in each drug. Data for double forebrain/brainstem KOs are derived from four mice withn=16 recording sites in con,n=7 sites in mec andn=9 sites in nic. All data are means±s.e.m. con, control conditions; mec, mecamylamine; nic, nicotine. Figure 5: Loss of brainstem-derived ACh does not affect local regulation of striatal DA release. ( a – d ) Voltammetric measurements of extracellular [DA] o in the CPu of striatal slices. ( a ) Representative single-pulse (1 p) and five-pulse (5 p) evoked [DA] o recorded in brainstem KO and forebrain/brainstem double KO mice. ( b , c ) Mean peak [DA] o evoked by 1 p and 5 p stimulation shows that DA release is not significantly altered in brainstem KO versus control mice ( b ). In double KO mice, there is a general suppression of DA release up to 10 Hz, maintenance of release levels at 25 and 50 Hz, and enhanced peak [DA] o at 100 Hz ( b ) (*** P <0.001 versus control; unpaired t -test for comparison of 1 p or two-way ANOVA with Bonferroni correction for comparison of 5 p). ( c ) Frequency dependence (5 p-to-1 p ratio) of evoked [DA] o in brainstem and double KO mice under control conditions (con) and in the presence of the nAChR antagonist mecamylamine (mec; 5 μM) or a desensitizing concentration of the nAChR agonist nicotine (nic; 500 nM) (*** P <0.001 mec versus con, ### P <0.001 nic versus con, two-way ANOVA with Bonferroni correction). The 1 p-to-5 p ratio in double KO mice under control conditions was indistinguishable from those seen in control mice in mec or nic ( P >0.05 for each frequency for either mec or nic, two-way ANOVA with Bonferroni correction). ( d ) 1 p evoked [DA] o in double KO mice was not suppressed by either mec or nic, in contrast to brainstem KO mice (*** P <0.001 versus con, one-way ANOVA with Dunnett’s correction). Data for brainstem KOs are derived from four mice with n =16 recording sites in con and n =8 sites in each drug. Data for double forebrain/brainstem KOs are derived from four mice with n =16 recording sites in con, n =7 sites in mec and n =9 sites in nic. All data are means±s.e.m. con, control conditions; mec, mecamylamine; nic, nicotine. Full size image Locomotor behaviour of ACh KO mice in a novel environment To test the behavioural consequences arising from the total loss of forebrain and or brainstem cholinergic regulation, we evaluated the locomotor behaviour of naive mice in the novel environment of the open field arena, which is linked to burst firing of DA neurons and consequent DA release [19] , [20] , [30] , [31] . Forebrain KO mice were hyperactive and hyperkinetic in that the total distance travelled during the first 10 min in the arena was significantly greater than that of non-mutant littermate control mice ( Fig. 6a ), and the movement velocity was enhanced ( Fig. 6b ). To assess the DA dependence of open field activity, we administered the competitive D2 receptor antagonist raclopride, whose displacement is commonly used as an index of DA release in human PET studies [32] , [33] . We found that raclopride was effective at suppressing total locomotor activity in forebrain KO mice, but only at a higher dose (>0.25 mg kg −1 ) than that necessary to decrease activity in control mice ( Fig. 6d ). The decreased efficacy of low-dose raclopride in forebrain KO mice argues against a role for increased receptor sensitivity from decreased tonic DA release as a contributing factor in the motor response. Instead, these data indicate elevated [DA] o at postsynaptic D2 receptors on striatal output neurons in these animals, when placed in a novel environment, and are consistent with the increase in phasic versus tonic striatal DA efflux observed in response to phasic stimulation in vitro ( Figs 2 and 3 ). 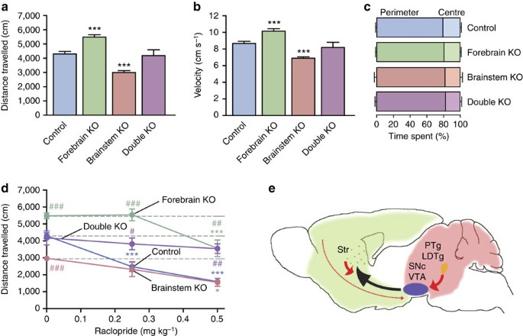Figure 6: Hyperactivity in forebrain ACh KO mice is normalized by D2R antagonism or by loss of brainstem ACh. (a,b) Summary of open field activity showing changes in total distance travelled per 10 min assay (a) and velocity of movement (b) in naive control (n=26), forebrain KO (n=12), brainstem KO (n=14) and forebrain/brainstem double KO (n=8) mice; ***P<0.001 versus control, one-way ANOVA with Dunnett’s correction. (c) Loss of brain ACh does not alter anxiety-related behaviour in the open field arena. There were no significant differences in the time spent in the centre versus perimeter zones during the first 10 min in the arena between non-mutant control (n=26), forebrain KO (n=12), brainstem KO (n=14) and forebrain/brainstem double KO (n=8) mice;P>0.05 versus control, one-way ANOVA with Dunnett’s correction. (d) Titration of raclopride dosage reveals the hyperdopaminergic phenotype of forebrain cholinergic mutants (n=4–12) versus control (n=5–26). Raclopride has little effect on locomotor activity when brainstem ACh is removed, suggesting lower D2 receptor activation in hypoactive brainstem KO mice (n=4–14) than in control mice. Double KO mice exhibit a similar insensitivity to raclopride to that seen in brainstem KO mice (n=6–8). *P<0.05; ***P<0.001 versus 0 mg kg−1in each mouse group, one-way ANOVA with Bonferroni correction;##P<0.01;###P<0.001 versus control mice, two-way ANOVA with Bonferroni correction. (e) Sagittal schematic depicting a model for coordinate regulation of DA release at the presynaptic level by striatal cholinergic interneurons (green territory) and at the soma by PTg/LDTg cholinergic projection neurons (red territory) as well as by descending forebrain projections from the prefrontal cortex, ventral pallidum and hippocampus (green territory). All data are means±s.e.m. Figure 6: Hyperactivity in forebrain ACh KO mice is normalized by D2R antagonism or by loss of brainstem ACh. ( a , b ) Summary of open field activity showing changes in total distance travelled per 10 min assay ( a ) and velocity of movement ( b ) in naive control ( n =26), forebrain KO ( n =12), brainstem KO ( n =14) and forebrain/brainstem double KO ( n =8) mice; *** P <0.001 versus control, one-way ANOVA with Dunnett’s correction. ( c ) Loss of brain ACh does not alter anxiety-related behaviour in the open field arena. There were no significant differences in the time spent in the centre versus perimeter zones during the first 10 min in the arena between non-mutant control ( n =26), forebrain KO ( n =12), brainstem KO ( n =14) and forebrain/brainstem double KO ( n =8) mice; P >0.05 versus control, one-way ANOVA with Dunnett’s correction. ( d ) Titration of raclopride dosage reveals the hyperdopaminergic phenotype of forebrain cholinergic mutants ( n =4–12) versus control ( n =5–26). Raclopride has little effect on locomotor activity when brainstem ACh is removed, suggesting lower D2 receptor activation in hypoactive brainstem KO mice ( n =4–14) than in control mice. Double KO mice exhibit a similar insensitivity to raclopride to that seen in brainstem KO mice ( n =6–8). * P <0.05; *** P <0.001 versus 0 mg kg −1 in each mouse group, one-way ANOVA with Bonferroni correction; ## P <0.01; ### P <0.001 versus control mice, two-way ANOVA with Bonferroni correction. ( e ) Sagittal schematic depicting a model for coordinate regulation of DA release at the presynaptic level by striatal cholinergic interneurons (green territory) and at the soma by PTg/LDTg cholinergic projection neurons (red territory) as well as by descending forebrain projections from the prefrontal cortex, ventral pallidum and hippocampus (green territory). All data are means±s.e.m. Full size image Considering that brainstem cholinergic inputs regulate the transition of midbrain DA neurons from tonic to burst firing modes [9] , we next examined the effects of removing these brainstem ACh signalling pathways on exploratory behaviour in the novel environment of the open field arena ( Fig. 6 ). Brainstem KO animals exhibited significantly less exploratory activity in the open field and were hypokinetic compared with control mice ( Fig. 6a ). As the removal of ChAT was restricted to the rostral brainstem, this hypoactivity was not due to loss of cholinergic activity from motor neurons in the hindbrain or spinal cord ( Fig. 4c ). These data are consistent with the expected decrease in phasic DA neuron firing with loss of brainstem cholinergic input. Indeed, raclopride had little effect on exploratory motor activity, even at the higher dose ( Fig. 6d ), thereby suggesting lower burst-driven D2 receptor activation in these animals than in control mice. Remarkably, the exploratory activity of animals lacking both forebrain- and brainstem-derived ACh was normalized to that of non-mutant control mice (mean distance travelled, P >0.05 versus control) ( Fig. 6a ), as was the velocity of movement ( P >0.05 versus control) ( Fig. 6b ). Thus, the enhanced phasic-to-tonic striatal DA release in these mice can compensate for the diminished burst output of midbrain DA neurons arising from the loss of brainstem cholinergic signalling, resulting in normal motor output. Consistent with a key role for burst-driven D2 receptor activation during exploration of a novel environment, double KO mice showed similar insensitivity to raclopride to that seen in brainstem KO animals ( Fig. 6d ). We did not find any difference across genotypes in the ratio of time spent in the centre versus perimeter zones of the open field arena during the 10 min of testing ( Fig. 6c ), indicating that anxiety-related behaviour changes were not a contributing factor to the differences in exploration observed across the genotypes. We show here that loss of forebrain ACh leads to increased phasic-to-tonic DA signalling throughout the striatal complex and hyperactivity in contexts that stimulate brainstem ACh activity and burst firing of DA neurons (for example, a novel environment), whereas loss of brainstem ACh leads to hypoactivity under similar conditions. Nevertheless, the striatum does not work in isolation, so that it is likely that the behaviour observed in our forebrain KOs is a synthetic phenotype arising from the total removal of forebrain ACh, with consequent alterations in the activities of descending glutamatergic projections from the prefrontal cortex, ventral pallidum and hippocampus that converge upon the SNc/VTA. Overall, our results support a model in which brainstem cholinergic inputs to midbrain DA neurons provide key regulation of the transition from tonic to burst firing modes that is then stimulated by diverse glutamatergic inputs [34] , with independent regulation of axonal DA release probability in the striatum by cholinergic interneurons signalling through nAChRs ( Fig. 6e ). A number of studies have examined the role of forebrain cholinergic neurons (striatal and projection) in regulating motor activity; however, to date the overall conclusion remains unclear. Complete loss of cholinergic cells in the NAc leads to hyperactivity [35] , whereas disruption of ACh neurotransmission via genetic ablation of the vesicular ACh transporter ( VAChT ) in all striatal interneurons does not change spontaneous locomotor activity [36] . Given that striatal cholinergic interneurons can co-release glutamate [37] , Guzman et al . [36] argue that the lack of change in locomotor activity is because glutamate release remains intact in this VAChT KO model. On the other hand, optogenetic inhibition of cholinergic interneurons in the CPu or NAc, which should prevent release of both ACh and glutamate, also has no effect on spontaneous locomotor behavior [38] , [39] . It is relevant to note that immunolesions of forebrain cholinergic projection neurons with 192 IgG-saporin (which spares striatal cholinergic interneurons) also fail to produce alterations in locomotion behaviour [40] . Our studies differ from this previous body of work in several ways. First, by targeting ChAT we examined the complete and selective loss of ACh, whereas disruption of VAChT leads to the accumulation of intracellular ACh [41] that could potentially result in residual cholinergic tone via non-quantal release mediated by the choline transporter [42] . Second, we deliberately examined motor behaviour in a novel environment, which leads to DA neuron burst firing and consequent DA release [19] , [20] , [30] , [31] . This novelty is lost in typical studies of locomotor behaviour that include an acclimation step [43] . Our data therefore refocus attention back on cholinergic regulation of striatal DA release as a component of motivated behaviour. The importance of these behavioural findings has been augmented by the recent demonstration that activation of striatal cholinergic interneurons directly trigger axonal DA release [11] , [12] . Our results in forebrain KO mice indicate that in the absence of local DA release regulation by striatal ACh in forebrain ChAT KO mice, the consequent absence of cholinergic gating of DA release leads to DA signalling that more faithfully reflects DA neuron activity. The simplest explanation for the hypoactive phenotype of brainstem KO mice is decreased phasic activity of midbrain DA neurons [9] ; however, other structures also receive cholinergic innervation from the PTg and LDTg, including the thalamus [44] . Given that the thalamus provides glutamatergic inputs to MSNs, reduction of cholinergic signalling within the thalamus could be a contributing factor to the hypoactivity phenotype observed. However, as thalamic input provides much less robust excitation of MSNs than does cortical input [45] , changes in thalamic activation alone should have only a minor direct effect on MSN output. Glutamatergic input from the thalamus can also activate striatal cholinergic interneurons [11] , [46] , although the net consequence of this on motor behaviour is difficult to predict. Thalamic activation can trigger striatal DA release via stimulation of local cholinergic interneurons and consequent activation of nAChRs on DA axons [11] , [46] , such that removal of brainstem cholinergic input to the thalamus could contribute to the hypoactivity seen in brainstem ACh KO mice via reduction of this pathway. On the other hand, thalamic activation of cholinergic interneurons can also decrease glutamatergic input to MSNs via mAChRs on cortical and thalamic terminals [46] , [47] , and enhance activation of indirect-pathway MSNs [15] , [46] , [48] , so that reduction of this process would be predicted to contribute to hyperactivity, which is opposite from what we observed in brainstem ACh KO mice. In addition to the thalamus, loss of brainstem cholinergic input to other brain regions might also contribute to the observed hypoactivity phenotype. General PTg lesion does lead to hypoactivity and to increased activity of the subthalamic nucleus and SN pars reticulata (SNr), however, these responses are thought to be secondary to the glutamatergic PTg inputs to SNc DA neurons [49] that would not be affected by brainstem ChAT removal. Strikingly, motor behaviour is normal in double KO mice, suggesting that any deficits in DA neuron burst firing from loss of brainstem cholinergic inputs is compensated by amplification of striatal phasic-to-tonic DA signalling in the absence of local cholinergic regulation. Behavioural normalization in double KOs also argues against a primary role for thalamic drive of cholinergic interneurons and consequent DA release in exploratory behaviour in a novel environment. The mice introduced here provide unique models to examine the role of ACh in a variety of behavioural contexts. Indeed, a major advantage of these mice is that they provide a reproducible and non-invasive means of selectively eliminating cholinergic activity in forebrain versus brainstem regions without loss of the cells themselves. This is important given that many of these neurons can also release other transmitters/modulators in addition to ACh that may impact brain physiology [37] . Thus, the selective removal of ACh synthesis achieved by our genetic methods provides a more specific means by which to examine the role of ACh in brain function and animal behaviour. The present findings highlight the critical role of forebrain and brainstem cholinergic signalling in regulating exploratory motor activity, and how imbalances in brain cholinergic tone can affect pathways that converge on dopaminergic circuits. The distinct differences in DA-dependent behaviours between forebrain and brainstem ACh KO mice and the normalization of motor behaviour in double KOs provides novel insights into ACh/DA interactions and the balance of ACh activities throughout the brain that is required for proper motor function. Mice and genotyping Mice harbouring a conditional (‘floxed’) allele for ChAT were obtained as a kind gift from Dr Joshua Sanes [21] . Genotyping by PCR for the wild-type ChAT allele was performed with the following primers: 5′-CAACCGCCTGGCCCTGCCAGTCAACTCTAG-3′ and 5′- GAGGATGAAATCCTGACAGATTCCAACAGG-3′. The ChAT flox allele was genotyped by PCR using the following primers: 5′-TGGTTCTTTCCGCCTCAGGACTCTTCCTTT-3′ and 5′-TAACCAAACGTAATATATGTTTGTTGGAGC-3′. The Nkx2.1 Cre BAC transgenic line [22] , a kind gift from Dr Stewart Anderson, was genotyped using the primers 5′-AAGGCGGACTCGGTCCACTCCG-3′ and 5′-TCGGATCCGCCGCATAACCAG-3′. The En1 Cre line [28] , a kind gift from Dr Alex Joyner, was genotyped using the primers 5′-GCCTTCTTCCTCTCCGCGCAC-3′ and 5′-TCGGATCCGCCGCATAACCAG-3′ (same reverse Cre primer as used with Nkx2.1 Cre genotyping). All experiments used heterozygous non-mutant transgenic littermates as controls (that is, Nkx2.1 Cre ; ChAT flox/+ , En1 Cre ; ChAT flox/+ , ChAT flox/flox and ChAT flox/+ are referred to as ‘control’ in the main text). We used these littermate controls rather than genuine wild-type ( ChAT +/+ ) animals to subtract out non-specific phenotypes that might arise from the presence of the Cre allele (for example, non-specific effects of Cre recombinase expression, or genomic alterations arising from transgene insertion) or ChAT flox allele (for example, potentially hypomorphic properties). It should be noted, however, that the expression pattern of ChAT mRNA as determined by in situ hybridization staining did not differ among the control genotypes. Moreover, levels of ACh should not be altered in these heterozygous control animals, as although ChAT enzymatic activity is essential for ACh production it is not the rate-limiting step, which is consistent with a lack of differences in voltammetric or behavioural data among these control groups. All animal handling procedures were in accordance with the National Institutes of Health guidelines and were approved by the Institutional Animal Care and Use Committees of New York University School of Medicine. In situ hybridization To generate an antisense cRNA in situ hybridization probe specific for the region flanked by loxP sites (exons 3–4), the following primers were used to generate a PCR template for probe synthesis (T7) from a full-length mouse ChAT cDNA clone (Open Biosystems clone ID: 40129512): 5′-GACTTACCTAAGTTGCCAGTG-3′ and 5′-AATTAATACGACTCACTATAGCTTAGCTGGTCATTGGTGT-3′. In situ hybridization with digoxigenin-labelled cRNA probes was performed essentially as previously described [50] . Briefly, sections (16–20 μm thick) were air dried, fixed in 4% paraformaldehyde in phosphate-buffered saline (PBS), pH 7.2 (PFA; 10 min at 4 °C), treated at room temperature sequentially with 1.5% H 2 O 2 in methanol (15 min), 0.2 M HCl (8 min), proteinase K (10 μg ml −1 PBS; 5 min), 4% PFA (10 min, 4 °C) and acetylation buffer (0.1 M triethanolamine, 0.045 N NaOH, 0.025% acetic anhydride), with PBS washes (3 × 5 min) between each step, before overnight hybridization at 55 °C (100 ng probe per millilitre buffer: 50% formamide, 10% dextran sulphate, 1% Denhardt’s solution, 250 μg ml −1 yeast tRNA, 0.3 M NaCl, 20 mM Tris–HCl pH 8.0, 5 mM EDTA, 10 mM NaH 2 PO 4 , 1% sarcosyl). Following hybridization, slides were washed in saline-sodium citrate buffer/50% formamide at 65 °C, treated with RNase (20 μg ml −1 in 0.5 M NaCl, 10 mM Tris–HCl, pH 7.5, 5 mM EDTA) and incubated overnight with anti-digoxigenin Fab fragments conjugated to peroxidase (Roche; 1:500 dilution in 100 mM maleic acid, 150 mM NaCl, 0.05% Tween-20, pH 7.5, with 1% blocking reagent). Following sequential incubations with biotinyl-tyramide and streptavidin-alkaline phosphatase, signal was visualized with standard nitro-blue tetrazolium and 5-bromo-4-chloro-3′-indolyl phosphate histochemistry. Hybridized sections were counterstained with Fast Red (Vector Labs), dehydrated, and coverslipped with Permount before imaging with a Zeiss Axioplan brightfield microscope. Voltammetric recording of DA release in striatal slices Procedures for preparing striatal slices and voltammetric recording of striatal DA release were according to those described previously [13] , [51] , [52] , [53] . Coronal forebrain slices (350 μm thick) were prepared from transgenic mice and their non-mutant control littermates (3–5 months of age) using a VT200S vibrating blade microtome (Leica Microsystems), then maintained in HEPES-buffered artificial cerebrospinal fluid (aCSF) at room temperature for at least 1 h before experimentation. Male mice were used for recordings in CPu whereas females were used for measurements in the NAc. For recording, slices were transferred to a submersion chamber (Warner Instruments LLC) maintained at 32 °C and superfused at 1.2 ml min −1 with bicarbonate-buffered aCSF containing (in mM): NaCl (124); KCl (3.7); NaHCO 3 (26); MgSO 4 (1.3); KH 2 PO 4 (1.3); glucose (10); and CaCl 2 (2.4), and saturated with 95% O 2 /5% CO 2 . After an equilibration period of at least 30 min, fast-scan cyclic voltammetry with carbon-fibre microelectrodes (7 μm diameter, 30–70 μm length, manufactured in-house) was used to monitor evoked [DA] o . Release of DA was elicited in either the dorsolateral portion of the striatum, the NAc core or the NAc shell using concentric bipolar stimulating electrodes placed on the surface of the slice ventromedially to the carbon fibre recording electrode. Voltammetric measurements were made using a Millar voltammeter (available by special request to Dr Julian Millar at St Bartholomew’s and the Royal London School of Medicine and Dentistry, University of London, UK). Scan range was −0.7 V to +1.3 V (versus Ag/AgCl), scan rate was 800 V s −1 , and the sampling interval was 100 ms. Data were acquired using a DigiData 200B A/D board controlled by Clampex 7.0 software (Molecular Devices). Released DA was identified according to voltammograms showing the single oxidation and reduction peak potentials that characterize the voltammetric signature of DA. To quantify evoked [DA] o , electrodes were calibrated with known concentrations of DA at 32 °C after each experiment in aCSF, in the presence and absence of each drug used during a given experiment. To decrease recording bias, the experimental design for the CPu typically involved sampling [DA] o in four recording sites of each striatal slice; two sites in control conditions and two sites in either mecamylamine (5 μM, Sigma) or nicotine (500 nM, Sigma). Two slices (one for each drug) were examined per mouse during an experimental day. In each recording site, release of DA was evoked by single-pulse (1 p) stimulation (0.4 to 0.6 mA amplitude, 0.1 ms duration) and by stimulation with five pulses (5 p) at 5, 10, 25, 50 and 100 Hz, applied at 5 min intervals. Stimulation frequencies were presented in either an ascending or descending order in the first control recording site and reversed for the second control site. The drug (either mecamylamine or nicotine) was then applied to the superfusing aCSF for at least 10–15 min before these patterns of stimulation were repeated for recording sites in the presence of drug. Experiments in the NAc core and shell were conducted in a similar manner to those described for the CPu only with two to four recording sites sampled in each NAc subregion of a single coronal slice in the absence of drugs. Open field behavioural assays Open field video recordings were performed in a 40 × 40cm white plexiglass arena using Noldus Ethovision Pro 3.1 tracking and analysis software. Naive experimental and control littermate male and female mice between 6 and 10 weeks of age were transferred in their respective home cages to the testing room at least 30 min before being placed in the clean arena. The first 10 min of activity were recorded for each mouse. We excluded one forebrain KO animal from the statistical analysis due to extreme hyperactivity. Raclopride (Sigma) in PBS was administered at the doses indicated by intraperitoneal injection 15 min before recording of animals in the open field arena. Data analysis Voltammetric DA recording: data are expressed as mean±s.e.m. where n indicates the number of recording sites in one to three slices from three to five mice per group and illustrated as either absolute [DA] o or the ratio of 5 p evoked [DA] o to 1 p. Open field activity recordings: data are expressed as mean±s.e.m., where n indicates the number of mice, and illustrated as total distance travelled and velocity of movement. Data were analysed using GraphPad Prism Software. Significance of differences was assessed using either an unpaired t -test, one-way ANOVA or two-way ANOVA as appropriate. Significance was considered to be P <0.05. How to cite this article: Patel, J.C. et al . Opposing regulation of dopaminergic activity and exploratory motor behavior by forebrain and brainstem cholinergic circuits. Nat. Commun. 3:1172 doi: 10.1038/ncomms2144 (2012).